Autonomous vascular networks synchronize GABA neuron migration in the embryonic forebrain Gamma-aminobutyric acid neurons, born in remote germinative zones in the ventral forebrain (telencephalon), migrate tangentially in two spatially distinct streams to adopt their specific positions in the developing cortex. The cell types and molecular cues that regulate this divided migratory route remains to be elucidated. Here we show that embryonic vascular networks are strategically positioned to fulfil the task of providing support as well as critical guidance cues that regulate the divided migratory routes of gamma-aminobutyric acid neurons in the telencephalon. Interestingly, endothelial cells of the telencephalon are not homogeneous in their gene expression profiles. Endothelial cells of the periventricular vascular network have molecular identities distinct from those of the pial network. Our data suggest that periventricular endothelial cells have intrinsic programs that can significantly mould neuronal development and uncovers new insights into concepts and mechanisms of central nervous system angiogenesis from both developmental and disease perspectives. Abnormalities in gamma-aminobutyric acid (GABA) neurons are implicated as a major factor in many neurological disorders ranging from epilepsy to autism and schizophrenia [1] , [2] , [3] , [4] . Whether this occurs by developmental and/or degenerative processes, abnormalities in neurons and their synapses usually receive prime consideration. However, when the key to complete understanding of the complicated pathophysiology as in the case of schizophrenia and finding solutions to successful therapy continues to elude us now for more than a century, it becomes critical to approach this problem with new perspectives. Our studies have shown the significance of the other cell type—‘endothelial cells’ in the embryonic forebrain and challenged notions of cerebral vascularization that imply that blood vessels sprout passively into the brain parenchyma from pial vascular plexuses to meet metabolic needs of growing neuronal populations [5] , [6] . Based on anatomical location, independent growth patterns and developmental regulation, telencephalic blood vessels fall into two categories: pial and periventricular. Although the neural tube directs the formation of the pial vessels that envelop it by embryonic day 9 (E9) (ref. 7 ), the periventricular vessels originate from a basal vessel on the telencephalic floor of the basal ganglia primordium and develop in an orderly, ventral-to-dorsal gradient by E11 (refs 5 , 6 ). The direction of the periventricular endothelial cell gradient matches the direction of GABA neuron migration from the basal to the dorsal telencephalon but with respect to timing, the angiogenesis gradient is in advance by about a day. GABA neurons on their tangential journey to the dorsal telencephalon arrive at the pallial–subpallial boundary (PSB) at E12 (Lopez-Bendito et al. [8] and Supplementary Fig. S1 ). Not only did the timing of this migration seem striking in comparison with the prior migration of endothelial cells of the periventricular network but also the periventricular endothelial cells (pv ecs) and GABA neurons follow the same migratory route. At E13, the distribution of GABA neurons into two spatially distinct streams in the dorsal telencephalon, a slender stream in the marginal zone (MZ) that is close to the pial network and another broader stream in the subventricular (SVZ) zone in the route of periventricular vessel gradient seemed very intriguing. The origins and routes of tangential migration of telencephalic GABA neurons are well established [9] , [10] , [11] . However, many missing links remain and the mechanisms that underlie GABA neuron tangential migration are not fully understood. Although, elegant work has demonstrated diverse modes of migration in the CNS, like radial-glial-dependent neuronal migration [12] , [13] and homophilic migration of the cells of the RMS [14] , the mode of migration of telencephalic GABA neurons has yet to be identified. For some time, it was speculated that GABA interneurons used the cortical-fugal fibres in the IZ as a guide [15] , [16] until it was conclusively ruled out [17] . The existing cortical radial-glial scaffold was also presumed to act as a guide for GABA interneurons when they enter the cortical plate [10] , however, no such glial guides are present when the GABA cells migrate out of the ventral telencephalon. The most widely accepted model for GABA neuron migration suggests that migration is dictated by the simultaneous activity of chemorepulsive and chemoattractive gradients [18] , [19] , [20] . Several families of ligands/receptors (Slit/Robo, semaphorin/neuropilin, Neuregulin-1/ErbB4 (refs 21 , 22 , 23 , 24 )), motogenic factors (HGF, SDF1(CXCL12), GDNF and BDNF (refs 20 , 25 , 26 , 27 , 28 , 29 ) as well as projection neuron precursors in the IZ-SVZ via CXCL12/CXCR4 signalling [30] have been proposed as candidates for guiding trajectories of GABA neurons. Nevertheless, key aspects into how exactly these factors influence formation and segregation of GABA neurons into a dual stream and direct them from the basal forebrain into the developing cortex remain undetermined and in this regard the enigma of GABA neuron tangential journey has remained elusive. Here we elucidate several new concepts about autonomy in embryonic vascular networks that regulate GABA neuron migration in the mouse telencephalon at an early embryonic stage, E13. We show that endothelial cells from the periventricular network are distinct from those of the pial network with remarkable versatility in being able to co-ordinate neuronal development. GABA neurons are closely associated with vascular networks From current literature [8] , [10] , [17] and from Supplementary Fig. S1 , the spatially distinct GABA neuron streams of the MZ and SVZ are obvious, but the telencephalic location, whether it is at the PSB or in the subpallium that GABA neurons seggregate to form these dual streams was unclear to us. Vibratome sections of E13 GAD65-GFP (green fluorescent protein) telencephalon were labelled with blood vessel marker, isolectin B4 at all rostro-caudal levels. Our observations reveal that formation of the dual GABA stream occurs deep within the ventral telencephalon. Indeed, GABA neurons can be visualized splitting into two streams in the ventral telencephalon and each stream enters one of two corridors created by the pial and periventricular networks ( Fig. 1a–j ). Confocal Z-stack images show us how the deep stream of GABA neurons taking this curved route are aligned with the periventricular vessel network. The rhombic vascular patterns en-sheath deep GABA neurons in a tube-like form ( Fig. 1c–j ). GABA neurons that segregate from the deep stream form the narrow superficial stream next to the pial network ( Fig. 1d–g ). The profile of periventricular vessels associated with the deep GABA neuron stream is directed tangentially towards the PSB ( Fig. 1a ). Periventricular vessels approaching the PSB have a slightly curved profile that extends into the pallium ( Fig. 1k , Supplementary Fig. S1 ). Periventricular vessels in the ganglionic eminence (GE) form a continuous tube-like plexus that connect to the vessels near the PSB ( Fig. 1k ). GABA neurons of the deep stream ( Fig. 1c–j ) and from the GE ( Fig. 1l ) adhere closely to their respective periventricular vascular profiles that lead them near the PSB where they form a single uniform stream ( Fig. 1l ). The profile of periventricular vessels near and around the PSB is very unique as it herds the GABA neuron stream uniformly into the SVZ of the dorsal telencephalon ( Fig. 1k ; Supplementary Fig. S1 ). This arrangement of periventricular vessel network in the ventral telencephalon that supports GABA neuron migration towards the PSB was observed in E13 slices at both rostral ( Fig. 1a–l ) and caudal levels ( Fig. 1m ). The lattice arrangement of periventricular vessels at the PSB ( Fig. 1o ) continues into the SVZ region of the dorsal telencephalon ( Fig. 1p ) where the deep stream of GABA neurons migrate ( Fig. 1q , Supplementary Fig. S1 ). We found a close physical association between the periventricular vascular network and deep stream of GABA neurons in both ventral and dorsal telencephalon ( Fig. 1a–t , Supplementary Fig. S1 ). This intimate vessel-GABA neuron contact was recapitulated in forebrain sections from E13 CD1 mice that were labelled with isolectin B4 and GAD65/GAD67 markers. High magnification images captured from ventral and dorsal telencephalon show processeses of GABA neurons wrapped around individual periventricular vessels ( Fig. 1u ). We quantified the association of vasculature-associated deep-seated GABA neurons in the telencephalon and found that nearly 84% of randomly selected GFP+ve cells were located within 5 μm of periventricular vessels ( Fig. 1w ). Interestingly, in the absence of a preformed periventricular vascular network in the dorsal telencephalon, GABA neurons from the ventral telencephalon failed to enter into the dorsal telencephalon ( Supplementary Fig. S2 ). 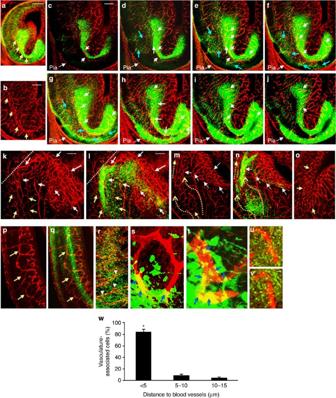Figure 1: GABA neurons are closely associated with vascular networks in the early embryonic telencephalon. (a) Surface view of an E13 GAD65-GFP telencephalon (vibratome section, 50 μm, coronal) labelled with isolectin B4. (b) Confocal image depicting vascular profile in the ventral telencephalon. Yellow arrows (a,b) point out tangential direction of periventricular vessels that support deep GABA neuron stream towards PSB. (c–j) The ventral telencephalon of the section in ‘a’ was studied by confocal microscopy. White arrows point to deep GABA neuron stream enwrapped in the periventricular network. Blue arrows point to GABA neurons segregating out to form the second stream close to the pial network. (k–n) Periventricular vascular profile close to PSB and in the GE (k) and the GABA neuron stream (l) associated with it at rostral (k,l) and caudal (m,n) levels. White dotted line marks PSB. Yellow arrows point out periventricular vascular profile leading towards PSB. White arrows points to the continuous plexus of periventricular vessels of the GE that connects to vessels near the PSB. Observe the vascular profile between the yellow dotted arrows (m,n) that channels GABA neurons towards PSB. (o) The lattice arrangement of periventricular vessels at the PSB continues into the SVZ region of the dorsal telencephalon (yellow arrows). (p,q) The periventricular vascular profile in the dorsal telencephalon (yellow arrows,p) and the deep stream of GABA neurons in close contact with the periventricular network (q). (r) The periventricular network is studded with GABA neurons (white arrowheads). (s–t) A magnified periventricular lattice (s) and vessel (t) showing intimate direct contact with GABA neurons (co-label in yellow, blue arrows). (u,v) Paraffin sections (20 μm) from E13 CD1 telencephalon were co-labelled with isolectin B4 (red) and GAD65/67 (green) markers. A × 40 magnification from ventral (u) and dorsal (v) telencephalon shows processes of GABA neurons wrapped around periventricular vessels. (w) Quantification of vasculature-associated GABA neurons in the telencephalon using ImageJ software. Data represent mean±s.d. (n=25, *P<0.0001, Student’st-test, group ‘<5 μm’ compared with group ‘<5–10 μm’). (a) Scale bar, 200 μm; (b) scale bar, 100 μm (appliesb–t); (u) scale bar, 50 μm (applies tov). Figure 1: GABA neurons are closely associated with vascular networks in the early embryonic telencephalon. ( a ) Surface view of an E13 GAD65-GFP telencephalon (vibratome section, 50 μm, coronal) labelled with isolectin B4. ( b ) Confocal image depicting vascular profile in the ventral telencephalon. Yellow arrows ( a , b ) point out tangential direction of periventricular vessels that support deep GABA neuron stream towards PSB. ( c – j ) The ventral telencephalon of the section in ‘ a ’ was studied by confocal microscopy. White arrows point to deep GABA neuron stream enwrapped in the periventricular network. Blue arrows point to GABA neurons segregating out to form the second stream close to the pial network. ( k – n ) Periventricular vascular profile close to PSB and in the GE ( k ) and the GABA neuron stream ( l ) associated with it at rostral ( k , l ) and caudal ( m , n ) levels. White dotted line marks PSB. Yellow arrows point out periventricular vascular profile leading towards PSB. White arrows points to the continuous plexus of periventricular vessels of the GE that connects to vessels near the PSB. Observe the vascular profile between the yellow dotted arrows ( m , n ) that channels GABA neurons towards PSB. ( o ) The lattice arrangement of periventricular vessels at the PSB continues into the SVZ region of the dorsal telencephalon (yellow arrows). ( p , q ) The periventricular vascular profile in the dorsal telencephalon (yellow arrows, p ) and the deep stream of GABA neurons in close contact with the periventricular network ( q ). ( r ) The periventricular network is studded with GABA neurons (white arrowheads). ( s – t ) A magnified periventricular lattice ( s ) and vessel ( t ) showing intimate direct contact with GABA neurons (co-label in yellow, blue arrows). ( u , v ) Paraffin sections (20 μm) from E13 CD1 telencephalon were co-labelled with isolectin B4 (red) and GAD65/67 (green) markers. A × 40 magnification from ventral ( u ) and dorsal ( v ) telencephalon shows processes of GABA neurons wrapped around periventricular vessels. ( w ) Quantification of vasculature-associated GABA neurons in the telencephalon using ImageJ software. Data represent mean±s.d. ( n =25, * P <0.0001, Student’s t -test, group ‘<5 μm’ compared with group ‘<5–10 μm’). ( a ) Scale bar, 200 μm; ( b ) scale bar, 100 μm (applies b – t ); ( u ) scale bar, 50 μm (applies to v ). Full size image Chemoattractive responses of GABA neurons are selective Given the formation of the dual GABA neuron stream in the ventral telencephalon and the close association of either stream with pial and periventricular vascular networks, it seemed inevitable that pial versus periventricular endothelial cell cues act in bringing about this segregation. We considered whether GABA neurons acquired information about their migration trajectories from guidance cues that they encountered in the endothelial cells en route . To answer these questions, our strategy was to present explants that derive GABA neurons of the deep stream and explants that derive GABA neurons of the superficial stream with a choice of pv ecs on one side and pial endothelial cells (pial ecs) on the other. Pial membranes were removed from intact telencephalon of E13 CD1 embryos by mechanical peeling and endothelial cells were isolated ( Fig. 2a ). The telencephalon without pial membranes was used to isolate pv ecs ( Fig. 2a ). Cultures of pial and pv ecs were thus prepared. We inserted culture inserts into the centre of 35 mm collagen-coated culture dishes to create a barrier and plated pv ecs on one side and pial ecs on the other ( Fig. 2b ). Cells were allowed to grow to confluence on either side of the barrier. The barrier was removed just at the start of the endothelial cell—GABA neuron co-culture experiment. Endothelial cells seated at the border at this stage could be observed forming a single line with no migration into the area that had been occupied by the barrier ( Fig. 2b ). Slice preparations of E13 GAD65-GFP brains were made and two explants were dissected out: (1) sub-cortical telencephalon containing GE and (2) subpial surface of ventral telencephalon (sps). Explants were placed in the centre of the endothelial cell-free area of culture dishes ( Fig. 2c ). This experimental design allowed us to sufficiently test chemoattractive activity of the deep and superficial set of GABA neurons when confronted with a choice of periventricular or pial ecs. Interestingly, GE explants were markedly attracted towards pv ecs and showed little response to pial ecs ( Fig. 2e ). An interesting observation was that a significant number of pv ecs lodged at the border at the start of the experiment crossed over and migrated towards the GE explant ( Fig. 2f ). A unique characteristic of pv ecs is their robust migratory capacity when compared with pial ecs ( Fig. 2f ). On the other hand, sps explants showed significant chemotactic response to pial ecs and minor response to pv ecs ( Fig. 2j ). Although many pv ecs migrated towards the explant ( Fig. 2k ), minimal response was seen on the part of the sps explant towards these endothelial cells ( Fig. 2l ). Co-labelled images of the chemoattractive response of GE and sps-derived GABA neurons towards periventricular and pial ecs are also shown ( Fig. 2o–r ). The chemoattractive response of GE and sps explants towards periventricular and pial ecs were quantified ( Fig. 2s ). The results of this experiment have been summarized in the schema ( Fig. 2u ). This experiment demonstrates that GABA neurons of the deep and superficial streams respond selectively to chemoattractive cues secreted by periventricular and pial ecs. 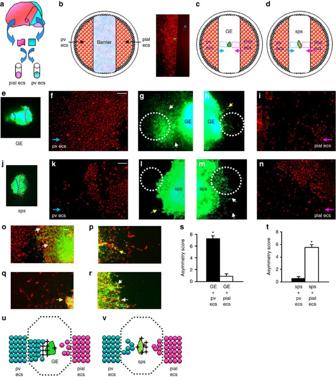Figure 2: Selective chemoattractive responses of GABA neurons towards pial and pv ecs. (a) Experiment schematic of isolation of pial and periventricular (pv) endothelial cells (ecs). (b) Diagram depicting preparation for chemoattractivity experiment. Isolectin B4 labelling (red) shows that ecs at barrier edge (green star) form a straight line with no escape into barrier occupied area (blue star) ensuring barrier reliability. (c,d) Schema of GE (dark green,c) and sps (light green,d) explants co-cultured with pv and pial ecs. Blue and pink dotted rectangles (c,d) depict areas of pv and pial ecs migration towards the explant in imagesf,i,kandn. Blue arrows (c,d) indicate direction of pv ecs migration (f,k) and pink arrows (c,d) indicate direction of pial ecs migration (i,n) towards the explant. (e–r) Robust chemoattractive activity in GE explant towards pv ecs only and significant chemoattractive activity in sps explant towards pial ecs only. Left half (black dots) of the explants (e,j) were magnified in g and l and right half (red dots) of the explants (e,j) were magnified inh,m. White dotted circles ing,h,l,mare magnified ino–rand depict co-labelling of neurons and ecs. Co-labelled images of the chemoattractive response of GE (o,p) and sps (q,r) derived GABA neurons towards pv (o,q) and pial (p,r) ecs. White arrows point to significant chemoattractive responses from explants (g,m,o,r) and yellow arrows point out little response from explants (h,l,p,q). (s,t) Quantification of chemoattraction of GE (s) and sps (t) explant towards pv and pial ecs; Data represent mean±s.d. (n=20, *P<0.0001, Student’st-test); scoring scheme applied from reference Flameset al.24. (u–v) Summary diagram fromc–t(n=20). Green stars depict chemoattractive activity from GE and sps explants, blue circles represent pv ecs and pink circles represent pial ecs. Robust migration of pv ecs towards GE explant was observed when compared to pial ecs. Robust chemoattractivity of GE explants to pv ecs only (u) and sps explants to pial ecs only (v). (f) Scale bar, 100 μm (applies also tog–i,k–n); (o)scale bar, 50 μm (applies also top–r). Figure 2: Selective chemoattractive responses of GABA neurons towards pial and pv ecs. ( a ) Experiment schematic of isolation of pial and periventricular (pv) endothelial cells (ecs). ( b ) Diagram depicting preparation for chemoattractivity experiment. Isolectin B4 labelling (red) shows that ecs at barrier edge (green star) form a straight line with no escape into barrier occupied area (blue star) ensuring barrier reliability. ( c , d ) Schema of GE (dark green, c ) and sps (light green, d ) explants co-cultured with pv and pial ecs. Blue and pink dotted rectangles ( c , d ) depict areas of pv and pial ecs migration towards the explant in images f , i , k and n . Blue arrows ( c , d ) indicate direction of pv ecs migration ( f , k ) and pink arrows ( c , d ) indicate direction of pial ecs migration ( i , n ) towards the explant. ( e – r ) Robust chemoattractive activity in GE explant towards pv ecs only and significant chemoattractive activity in sps explant towards pial ecs only. Left half (black dots) of the explants ( e , j ) were magnified in g and l and right half (red dots) of the explants ( e , j ) were magnified in h , m . White dotted circles in g , h , l , m are magnified in o – r and depict co-labelling of neurons and ecs. Co-labelled images of the chemoattractive response of GE ( o , p ) and sps ( q , r ) derived GABA neurons towards pv ( o , q ) and pial ( p , r ) ecs. White arrows point to significant chemoattractive responses from explants ( g , m , o , r ) and yellow arrows point out little response from explants ( h , l , p , q ). ( s , t ) Quantification of chemoattraction of GE ( s ) and sps ( t ) explant towards pv and pial ecs; Data represent mean±s.d. ( n =20, * P <0.0001, Student’s t -test); scoring scheme applied from reference Flames et al. [24] . ( u – v ) Summary diagram from c – t ( n =20). Green stars depict chemoattractive activity from GE and sps explants, blue circles represent pv ecs and pink circles represent pial ecs. Robust migration of pv ecs towards GE explant was observed when compared to pial ecs. Robust chemoattractivity of GE explants to pv ecs only ( u ) and sps explants to pial ecs only ( v ). ( f ) Scale bar, 100 μm (applies also to g – i , k – n ); ( o) scale bar, 50 μm (applies also to p – r ). Full size image Endothelial cells selectively guide GABA neuron migration To test if distinct endothelial cells could specifically influence the migration of GABA neurons, we evaluated the migration of deep and superficial sets of GABA neurons from GE and sps explants on thin layers of basement membrane (BM) matrices that was seeded with either periventricular, pial or control endothelial cells ( Fig. 3a–i ). Control endothelial cells were prepared from other embryonic brain regions (E13 mesencephalon and metencephalon combined). GE explants showed significantly more robust migration on matrices seeded with pv ecs, both in terms of cell number and migratory distance when compared with explants cultured on matrices seeded with pial or control endothelial cells ( Fig. 3b–e ). On the other hand, sps explants migrated significantly on matrices seeded with pial ecs when compared with periventricular or control endothelial cells ( Fig. 3f–i ). The controls ( Fig. 3d ) confirm that the effects on cell migration from GE and sps explants are specific for pv ecs and pial ecs ( Fig. 3b–i ). As the BM matrix itself might be a conducive substrate for migration, we cultured our explants on a bed of pial, periventricular or control endothelial cells alone. Our results were similar to those obtained on BM matrices. GABA neurons from sps explants migrated well only on pial ecs ( Fig. 3j ) and GABA neurons from GE explants migrated extensively only on pv ecs ( Fig. 3k ). In some of our culture dishes, pv ecs formed lattice patterns and the close association of migrating GABA neurons to these endothelial cells closely resembled the in vivo situation ( Fig. 3l ). Even within 6 h, GABA neurons from GE explants were seen taking a migratory route in close association to pv ecs ( Fig. 3m–o ). These results show that pv ecs selectively promote migration of the deep GABA neuron population while pial ecs promote migration of the superficial GABA neuron population. 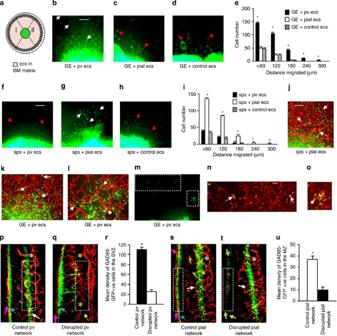Figure 3: Endothelial cells provide cues for selective sorting and migration of individual streams of GABA neurons. (a) Experiment schematic: either pv, pial or control ecs were seeded in BM matrix and cell migration from GE or sps explants was analysed in sectors I and II. (b–i) Robust migration of GE-derived cells in response to pv ecs compared with pial and control ecs (b–e) and robust migration of sps-derived cells in response to pial ecs compared with pv and control ecs (f–i). White arrows point to robust migration and red arrows point to little migration. (e,i) Quantification of migration assays inb–dandf–h, respectively. (n=25, mean±s.d., *P<0.0001, Student’st-test.) (j,k) Robust migration (white arrows) of cells from sps explants (j) and GE explants (k) when cultured on pial ecs (j) and pv ecs (k), respectively. (l) Sometimes migration of GFP+ve cells on pv ecs (white arrows) recapitulatedin vivosituation. (m–o) Migration of GFP+ve cells from GE explants when cultured with pv ecs within 6 h. Dotted rectangles from ‘m’ have been highlighted in ‘n’ and ‘o’ as co-labelled images. White arrows (n,o) indicate close contact of migratory cells with pv ecs. (p–u) Disruption of pv network (yellow stars,q) resulted in significant reduction of SVZ stream (yellow arrow,q) when compared with the respective control (p) while the MZ stream was unaffected (q) and disruption of pial network (green arrows,t) resulted in significant reduction of the MZ stream (yellow arrow,t) while the SVZ stream was unaffected (t). White arrows (p,s,t) point to normal SVZ streams. Blue arrows (p,q,s) point to normal MZ stream and pink arrows (p,q,s) depicts continuous pial network. White stars (p,s,t) depict normal periventricular network. White dotted box (p,q,s,t) was the area selected for cell counts. (r,u) Quantification of GAD65-GFP+ve cells in control and disrupted pv (p,q) and pial (s,t) network slices (n=25, mean±s.d., *P<0.001, Student’st-test). (b) Scale bar, 100 μm (applies also toc,d,f–h,j–m,p,q,s,t); (n) scale bar, 50 μm (applies also to ‘o’). Figure 3: Endothelial cells provide cues for selective sorting and migration of individual streams of GABA neurons. ( a ) Experiment schematic: either pv, pial or control ecs were seeded in BM matrix and cell migration from GE or sps explants was analysed in sectors I and II. ( b – i ) Robust migration of GE-derived cells in response to pv ecs compared with pial and control ecs ( b – e ) and robust migration of sps-derived cells in response to pial ecs compared with pv and control ecs ( f – i ). White arrows point to robust migration and red arrows point to little migration. ( e , i ) Quantification of migration assays in b – d and f – h , respectively. ( n =25, mean±s.d., * P <0.0001, Student’s t -test.) ( j , k ) Robust migration (white arrows) of cells from sps explants ( j ) and GE explants ( k ) when cultured on pial ecs ( j ) and pv ecs ( k ), respectively. ( l ) Sometimes migration of GFP+ve cells on pv ecs (white arrows) recapitulated in vivo situation. ( m – o ) Migration of GFP+ve cells from GE explants when cultured with pv ecs within 6 h. Dotted rectangles from ‘ m ’ have been highlighted in ‘ n ’ and ‘ o ’ as co-labelled images. White arrows ( n , o ) indicate close contact of migratory cells with pv ecs. ( p – u ) Disruption of pv network (yellow stars, q ) resulted in significant reduction of SVZ stream (yellow arrow, q ) when compared with the respective control ( p ) while the MZ stream was unaffected ( q ) and disruption of pial network (green arrows, t ) resulted in significant reduction of the MZ stream (yellow arrow, t ) while the SVZ stream was unaffected ( t ). White arrows ( p , s , t ) point to normal SVZ streams. Blue arrows ( p , q , s ) point to normal MZ stream and pink arrows ( p , q , s ) depicts continuous pial network. White stars ( p , s , t ) depict normal periventricular network. White dotted box ( p , q , s , t ) was the area selected for cell counts. ( r , u ) Quantification of GAD65-GFP+ve cells in control and disrupted pv ( p , q ) and pial ( s , t ) network slices ( n =25, mean±s.d., * P <0.001, Student’s t -test). ( b ) Scale bar, 100 μm (applies also to c , d , f – h , j – m , p , q , s , t ); ( n ) scale bar, 50 μm (applies also to ‘ o ’). Full size image To study the importance of either vascular network for the formation of deep and superficial GABA neuron streams, we selectively disrupted either the periventricular vessel gradient ( Fig. 3p–r ) or the pial network ( Fig. 3s–u ). Cultures of intact E12 GAD65-GFP telencephalon were prepared (the stage when GABA neurons have just arrived at the PSB) and beads treated with angiogenesis inhibitor TNP-470, a fumagillin derivative [31] , [32] , were placed along the ventricular zone of the dorsal telencephalon. By this method, we were able to disrupt the periventricular vessel gradient selectively while the pial network was unaffected ( Fig. 3q ). The concentration of angiogenesis inhibitor used in this experiment does not cause cell death of cultured GABA neurons or affect migration from explant cultures ( Supplementary Fig. S3 ). Control explants received beads treated with PBS and showed normal formation of periventricular and pial networks and the dual streams of GABA neurons ( Fig. 3p ). Interestingly, in the absence of a normal periventricular vessel network, formation of the deep stream in the SVZ was significantly affected, while the superficial stream in the MZ formed adjacent to the pial network ( Fig. 3q ). As meningeal cells rapidly degenerate upon exposure to 6-hydroxydopamine (ref. 5 ), we exposed E12 GAD65-GFP telencephalic explants to 6-hydroxydopamine. In explants treated with 6-hydroxydopamine, although pial network was disrupted, periventricular vessels were unaffected ( Fig. 3t ). Disruption of the pial network significantly disturbed superficial stream formation in the MZ ( Fig. 3t ) when compared with the respective control ( Fig. 3s ) while the deep stream of GABA neurons formed normally in the SVZ ( Fig. 3s ). The reduction in mean density of GABA neurons of the SVZ ( Fig. 3p ) and MZ ( Fig. 3s ) streams were quantified. Collectively these data point to a novel role for pial and periventricular vascular networks in instructing and promoting the selective migration of GABA neurons as two distinct streams in the early embryonic telencephalon. Unique gene expression in pv ecs As pial and pv ecs were independently capable of acting as substrates and providing distinct guidance cues to aid migration of the individual GABA neuron streams, we reasoned that the outcome of gene expression profiles of pial ecs and pv ecs would be distinct. To address this question, endothelial cells from pial, periventricular and control (mesencephalon and metencephalon combined) samples obtained from E13 Tie2-GFP mice (in which endothelial cells express GFP) were stringently sorted by dual FACS analysis (with an endothelial cell marker, CD31) to obtain pure populations of pial, periventricular and control endothelial cells, respectively ( Fig. 4a ). RNA was extracted from all samples and subsequent microarray hybridization and analysis were performed. 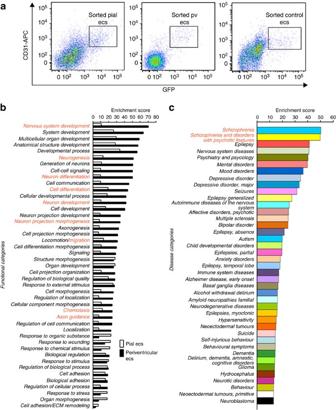Figure 4: Gene expression profile in pv ecs and its significance for brain development and disease. (a) Dual FACS analysis of pial samples (left panel), periventricular samples (middle panel) and control samples (right panel) from E13 Tie2-GFP embryos (n=70). The purity of sorted endothelial cell samples were ensured by collection of cells that were double positive for GFP and CD31. (b) A comparison of developmental processes’ categories that were enriched in pial and pv ecs. Some of the functional categories that represent critical developmental processes where pv ecs might have hereto unexplored roles have been highlighted (red). (c) Periventricular angiogenesis and disease: A classification of genes expressed in pv ecs that were particularly enriched in several psychiatric and neurological disease categories. Schizophrenia topped the list followed closely by epilepsy. Figure 4: Gene expression profile in pv ecs and its significance for brain development and disease. ( a ) Dual FACS analysis of pial samples (left panel), periventricular samples (middle panel) and control samples (right panel) from E13 Tie2-GFP embryos ( n =70). The purity of sorted endothelial cell samples were ensured by collection of cells that were double positive for GFP and CD31. ( b ) A comparison of developmental processes’ categories that were enriched in pial and pv ecs. Some of the functional categories that represent critical developmental processes where pv ecs might have hereto unexplored roles have been highlighted (red). ( c ) Periventricular angiogenesis and disease: A classification of genes expressed in pv ecs that were particularly enriched in several psychiatric and neurological disease categories. Schizophrenia topped the list followed closely by epilepsy. Full size image This resulted in 2,426 genes upregulated in pv ecs and 1,567 genes downregulated when compared with pial ecs. To examine the overall differences in expression closely, genes were classified into 45 functional categories ( Fig. 4b ). Interestingly, pv ecs showed increased expression in genes that are specific to the central theme of embryonic forebrain development like neurogenesis, differentiation, morphogenesis, migration, chemotaxis and axon guidance when compared with pial ecs. We screened for pathways and processes that were over- or under-represented in one endothelial cell type with respect to the other ( Supplementary Figs S4–S11 ). Gene expressions for biological processes and canonical maps containing genes controlling neuronal development, cell proliferation, cell migration and immune response were enriched in pv ecs ( Supplementary Figs S4–S7 ). Gene expressions for endothelial cell contacts by non-junctional mechanisms, chemokines and cell adhesion as well as extracellular matrix remodelling were comparable in pial versus pv ecs ( Supplementary Figs S8–S10 ). We next classified the genes according to disease categories and made another key discovery. The genes expressed in pv ecs were enriched in disease categories like schizophrenia, nervous system diseases, epilepsy, autism, mood and depressive disorders ( Figs 4c and 5a ), whereas those in pial ecs were enriched in inflammation and pathological process categories ( Fig. 5a ). Independent repeats of microarray hybridization and analysis performed with control endothelial cells and telencephalic pv ecs showed similar results. The genes expressed in pv ecs remained consistently enriched in disease categories like schizophrenia, psychiatric diseases, nervous system diseases, epilepsies, autism, bipolar, mood and depressive disorders when compared with control endothelial cells ( Fig. 5b ). The genes expressed in control endothelial cells were enriched in disease categories that were non neuro-psychiatric ( Fig. 5b ). This gene expression profile with enrichment of several neuro-psychiatric disease categories is thus a unique characteristic of pv ecs of the embryonic forebrain. As schizophrenia topped the list of disease categories, we identified some of the top common genes that were enriched in this category in pv ecs after comparisons with both pial and control endothelial cells ( Supplementary Data 1 ). In diseases like schizophrenia, epilepsy and autism, abnormalities have been widely reported in GABA neurons [3] , [4] , [33] , with increasing evidence that this may be in part due to incorrect differentiation and misguided migration of GABA neurons during brain development [34] , [35] . Interestingly, in our screen we found many genes commonly known to be expressed and/or traditionally believed to be confined to GABA neurons/interneurons and their precursors were expressed/upregulated in pv ecs ( Supplementary Table S1 ) and some in pial ecs ( Supplementary Table S2 ). Some of the top genes were subdivided into categories like transcription factors, cell-surface molecules essential for migration and genes related to ionic regulation that are involved in GABA signalling ( Supplementary Tables S1 and S2 ). For validation of differentially expressed genes, quantitative real-time PCR was performed on eight randomly picked genes, Gabrb3 , Gabra1 , Cxcr4 , Cdk5r1 , Foxg1 and Sez6l2c ( Fig. 5c ). Each of these genes were several fold upregulated in pv ecs ( Fig. 5c ). 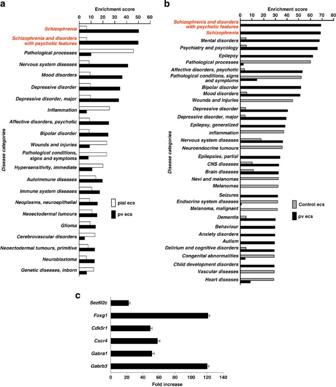Figure 5: Periventricular angiogenesis and disease. (a) A classification of disease categories that were enriched in pial and pv ecs. Schizophrenia (highlighted in red) topped the disease category enriched in pv ecs. (b) A classification of disease categories that were enriched in control and pv ecs. Schizophrenia (highlighted in red) topped the disease category enriched in pv ecs. (c) A subset of genes believed to be expressed/traditionally confined to GABA neurons, interneurons and their precursors that were enriched in pv ecs when compared with pial ecs in the microarray screen were validated by quantitative real-time PCR (mean±s.d.). Figure 5: Periventricular angiogenesis and disease. ( a ) A classification of disease categories that were enriched in pial and pv ecs. Schizophrenia (highlighted in red) topped the disease category enriched in pv ecs. ( b ) A classification of disease categories that were enriched in control and pv ecs. Schizophrenia (highlighted in red) topped the disease category enriched in pv ecs. ( c ) A subset of genes believed to be expressed/traditionally confined to GABA neurons, interneurons and their precursors that were enriched in pv ecs when compared with pial ecs in the microarray screen were validated by quantitative real-time PCR (mean±s.d.). Full size image Endothelial GABA A receptors modulate GABA neuron migration GABA A receptors are traditionally believed to be confined to GABA neurons, but our microarray and real-time PCR data detected high expression of these receptors in pv ecs ( Supplementary Table S1 ; Fig. 5c ) signifying that telencephalic angiogenesis has its own intrinsic GABA-signalling mechanism. GABA and its receptors-mediated signalling have been suggested to modulate progenitor cell proliferation, neuronal migration and circuit formation in the cortex [36] , [37] , [38] . Defects in GABA A receptor regulation has been suggested as a mechanism contributing to schizophrenia, epilepsy and autism [39] , [40] , [41] . Although there are reports of presence of GABA A receptors on blood vessel membranes, atria, left ventricle, descending aorta and in the endothelium lining of the vasculature of brain [42] , [43] , GAD immunoreactivities in endothelial cells of cerebral arteries [44] , GAD65 expression by in situ hybridization in cardiac arteries and major blood vessels of E12.5 embryo [45] , its functional significance remains unknown. Therefore, we selected one of the validated genes in pv ecs, GABA A receptor, Gabrb3 , associated with pyschiatric and neurodevelopmental disorders [2] , [46] , [47] , [48] , [49] , [50] , [51] to test its autonomous role in pv ecs. Co-labelling with isolectin B4 and GABRB3 antibodies showed robust expression of GABRB3 in pv ecs ( Fig. 6a ). GFP+ve endothelial cells from Tie2-GFP mouse brains confirmed GABRB3 expression in pv ecs ( Fig. 6c ). When GABRB3 expression was downregulated in pv ecs by small interfering RNA (siRNA) technique ( Fig. 6d ), there was a marked decrease in endothelial cell proliferation ( Fig. 6e ) confirming its role in periventricular angiogenesis. Subsequently, GE explants showed a lack of chemoattraction towards Gabrb3 siRNA-transfected endothelial cells when compared with the respective control ( Fig. 6f–i ). In addition, loss-of-function of Gabrb3 in pv ecs significantly decreased cell migration from GE explants ( Fig. 6j ) alone. As sps cells do not migrate on pv ecs ( Fig. 3f ), the migratory response of sps cells on control and siRNA-transfected ecs remained comparable ( Fig. 6k ) Thus, Gabrb3 siRNA-transfected pv ecs were unable to provide chemoattractive and guidance cues that are needed for GABA neuron migration. Interestingly, loss-of-function of GABRB3 downregulated GABA expression in pv ecs when compared with the respective control ( Fig. 6l–o ). GABA is known to act as a chemoattractant, providing directional cues to migrating neurons and enhancing chemotaxis or chemokinesis in the developing telencephalon [37] , [38] , [52] , [53] , [54] . Hence, we investigated for detection of secreted GABA by ELISA from control and Gabrb3 siRNA-transfected pv ecs. Although control siRNA-transfected pv ecs secreted GABA, in sharp contrast, GABA secretion was abolished from Gabrb3 siRNA-transfected pv ecs ( Fig. 6p ). 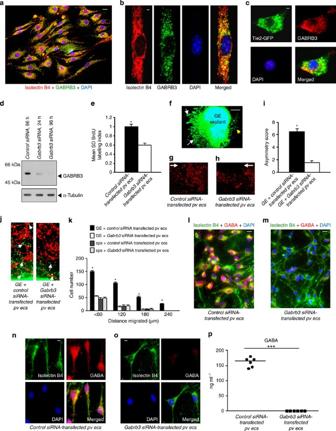Figure 6: Autonomous roles of GABAAreceptors in periventricular angiogenesis that influences deep GABA neuron populations. (a) A low magnification co-labelled image of isolectin B4, GABRB3 and DAPI labelling of pv ecs. (b) Individual isolectin B4, GABRB3, DAPI and co-labelled image of a pv ec ( × 60). (c) GFP, GABRB3, DAPI and merged image of a pv ec from Tie2-GFP telencephalon ( × 40). (d) Virtually complete knockdown of GABRB3 in pv ecs after 96 h ofGabrb3siRNA-transfection versus control transfections. α-tubulin was used as a loading control. (e) BrdU labelling indices were significantly decreased (n=20, mean±s.d., *P<0.001, Student’st-test) inGabrb3siRNA-transfected pv ecs when compared with control siRNA-transfected pv ecs. (f) GE explants showed marked chemoattraction (white arrows) to control siRNA-transfected pv ecs and this chemoattractive activity was significantly reduced (yellow arrow) towardsGabrb3siRNA-transfected pv ecs. (g,h) Migration of control (g) andGabrb3(h) siRNA-transfected pv ecs towards GE explant. Arrows show direction of ecs migration towards explant. (i) Quantification of attraction of GE cells towards control andGabrb3siRNA-transfected pv ecs (n=25, mean±s.d., *P<0.001, Student’st-test). (j) Cell migration from GE explants was significantly decreased when cultured onGabrb3siRNA- transfected pv ecs when compared with control siRNA-transfected pv ecs. White arrows point to cell migration from explant. (k) Quantification of migration assays of GE and sps explants on control andGabrb3siRNA-transfected pv ecs. Plot shows average±s.d. (n=20, *P<0.0001, Student’st-test, group ‘GE+control siRNA-transfected pv ecs’ compared with group ‘GE+Gabrb3siRNA-transfected pv ecs’). (l,m) Co-labelled images of isolectin B4, GABA and DAPI labelling of control (l) andGabrb3(m) siRNA-transfected pv ecs after 96 h. (n,o) Individual isolectin B4, GABA and DAPI labelling of control (n) andGabrb3(o) siRNA-transfected pv ecs and merged images at × 60 magnification. (p)Gabrb3siRNA-transfected pv ecs failed to secrete GABA in contrast to control siRNA-transfected pv ecs (n=6, mean±s.d., ***P<0.001, Student’st-test). (a) Scale bar, 50 μm (applies also tol,m); (b) scale bar, 15 μm (applies also toc,n,o); (f) scale bar, 100 μm (applies tog,h,j). Figure 6: Autonomous roles of GABA A receptors in periventricular angiogenesis that influences deep GABA neuron populations. ( a ) A low magnification co-labelled image of isolectin B4, GABRB3 and DAPI labelling of pv ecs. ( b ) Individual isolectin B4, GABRB3, DAPI and co-labelled image of a pv ec ( × 60). ( c ) GFP, GABRB3, DAPI and merged image of a pv ec from Tie2-GFP telencephalon ( × 40). ( d ) Virtually complete knockdown of GABRB3 in pv ecs after 96 h of Gabrb3 siRNA-transfection versus control transfections. α-tubulin was used as a loading control. ( e ) BrdU labelling indices were significantly decreased ( n =20, mean±s.d., * P <0.001, Student’s t -test) in Gabrb3 siRNA-transfected pv ecs when compared with control siRNA-transfected pv ecs. ( f ) GE explants showed marked chemoattraction (white arrows) to control siRNA-transfected pv ecs and this chemoattractive activity was significantly reduced (yellow arrow) towards Gabrb3 siRNA-transfected pv ecs. ( g , h ) Migration of control ( g ) and Gabrb3 ( h ) siRNA-transfected pv ecs towards GE explant. Arrows show direction of ecs migration towards explant. ( i ) Quantification of attraction of GE cells towards control and Gabrb3 siRNA-transfected pv ecs ( n =25, mean±s.d., * P <0.001, Student’s t -test). ( j ) Cell migration from GE explants was significantly decreased when cultured on Gabrb3 siRNA- transfected pv ecs when compared with control siRNA-transfected pv ecs. White arrows point to cell migration from explant. ( k ) Quantification of migration assays of GE and sps explants on control and Gabrb3 siRNA-transfected pv ecs. Plot shows average±s.d. ( n =20, * P <0.0001, Student’s t -test, group ‘GE+control siRNA-transfected pv ecs’ compared with group ‘GE+ Gabrb3 siRNA-transfected pv ecs’). ( l , m ) Co-labelled images of isolectin B4, GABA and DAPI labelling of control ( l ) and Gabrb3 ( m ) siRNA-transfected pv ecs after 96 h. ( n , o ) Individual isolectin B4, GABA and DAPI labelling of control ( n ) and Gabrb3 ( o ) siRNA-transfected pv ecs and merged images at × 60 magnification. ( p ) Gabrb3 siRNA-transfected pv ecs failed to secrete GABA in contrast to control siRNA-transfected pv ecs ( n =6, mean±s.d., *** P <0.001, Student’s t -test). ( a ) Scale bar, 50 μm (applies also to l , m ); ( b ) scale bar, 15 μm (applies also to c , n , o ); ( f ) scale bar, 100 μm (applies to g , h , j ). Full size image As Gabra2 was the only GABA A receptor identified from our microarray screen in pial ecs ( Supplementary Table S2 ), we tested if it might have a role in pial angiogenesis. Expression of GABRA2 in pial ecs was confirmed by co-labelling with isolectin B4 and GABRA2 antibodies ( Fig. 7a ). Pial ecs from Tie2-GFP mouse brains revealed GABRA2 expression ( Fig. 7c ). Downregulation of GABRA2 expression in pial ecs ( Fig. 7d ) resulted in a significant decrease in endothelial cell proliferation ( Fig. 7e ) confirming its role in pial angiogenesis. A decrease in chemoattractive response of sps explants towards Gabra2 siRNA-transfected pial ecs was observed ( Fig. 7f–i ). Cell migration from sps explants was significantly decreased on substrates of Gabra2 siRNA-transfected pial ecs when compared with the respective control ( Fig. 7j ). Cells from GE explants showed reduced migration on pial endothelial cell substrates whether they were transfected with control siRNA (similar to our observations in Fig. 3c ) or Gabra2 siRNA ( Fig. 7k ). Thus, Gabra2 siRNA-transfected pial ecs were unable to provide the necessary cues required by superficial GABA neurons. Furthermore, downregulation of GABRA2 significantly decreased GABA expression in pial ecs when compared with the respective control ( Fig. 7l–o ). Interestingly control pial ecs secreted GABA ( Fig. 7p ) at approximately twofold higher levels than control pv ecs ( Fig. 6p ). Gabra2 siRNA-transfected pial ecs failed to secrete GABA ( Fig. 7p ) similar to Gabrb3 siRNA-transfected pv ecs ( Fig. 6p ). Our results not only depict a new vascular source of GABA in the early embryonic telencephalon but also suggest that deep GABA neurons respond to low levels of GABA secreted by pv ecs and superficial GABA neurons respond to higher levels of GABA secreted by pial ecs ( Fig. 7q ). Our data signify a novel mechanism of endothelial cell-mediated seggregation and migration of GABA neurons in the embryonic telencephalon. 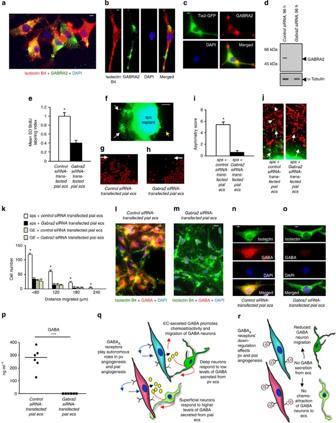Figure 7: Autonomous roles of GABAAreceptors in pial angiogenesis that influences superficial GABA neuron populations. (a,b) A low magnification co-labelled image of isolectin B4, GABRA2 and DAPI labelling of pial ecs. (b) Isolectin B4, GABRA2 and DAPI labelling of a pial ec ( × 48). (c) GFP, GABRA2 and DAPI labelling of a pial ec ( × 23). (d) Complete knockdown of GABRA2 in pial ecs after 96 h ofGabra2siRNA-transfection versus control transfections. α-Tubulin was used as loading control. (e) BrdU labelling indices were significantly decreased inGabra2siRNA-transfected pial ecs (n=20, mean±s.d., *P<0.001, Student’st-test). (f) sps explants showed chemoattraction (white arrows) to control siRNA-transfected pial ecs and this chemoattraction was reduced (yellow arrow) towardsGabra2siRNA-transfected pial ecs. (g,h) Migration of control (g) andGabra2(h) siRNA-transfected pial ecs towards sps explant. Arrows show direction of migration. (i) Quantification of sps explant chemoattraction towards control andGabra2siRNA-transfected pial ecs (n=25, mean±s.d., *P<0.0001, Student’st-test). (j) Cell migration from sps explants was decreased when cultured onGabra2siRNA-transfected pial ecs. White arrows illustrate cell migration. (k) Quantification of migration assays of GE and sps explants on control andGabra2siRNA-transfected pial ecs (n=20, mean±s.d., *P<0.0001, Student’st-test, group ‘sps+control siRNA-transfected pial ecs’ compared with group ‘sps+Gabra2siRNA-transfected pial ecs’). (l,m) Co-labelled images of isolectin B4, GABA and DAPI labelling of control (l) andGabra2(m) siRNA-transfected pial ecs. (n,o) Individual isolectin B4, GABA and DAPI labelling of control (n) andGabra2(o) siRNA-transfected pial ecs ( × 60). (p)Gabra2siRNA-transfected pial ecs failed to secrete GABA in contrast to control siRNA-transfected pial ecs (n=6, mean±s.d., ***P<0.001, Student’st-test). (q–r) Schema of GABAAreceptors-GABA signaling in pv ecs (blue) and pial ecs (pink) that has consequences for deep (dark green) and superficial (light green) GABA neuron populations. GABAAreceptors depicted as black ‘Y’ and GABA as yellow circles. (a) Scale bar, 40 μm; (b) scale bar, 13 μm; (c) scale bar, 28 μm; (f) scale bar, 100 μm (applies tog,h,j); (l) scale bar, 50 μm (applies also tom); and (n) scale bar, 15 μm (applies also too). Figure 7: Autonomous roles of GABA A receptors in pial angiogenesis that influences superficial GABA neuron populations. ( a , b ) A low magnification co-labelled image of isolectin B4, GABRA2 and DAPI labelling of pial ecs. ( b ) Isolectin B4, GABRA2 and DAPI labelling of a pial ec ( × 48). ( c ) GFP, GABRA2 and DAPI labelling of a pial ec ( × 23). ( d ) Complete knockdown of GABRA2 in pial ecs after 96 h of Gabra2 siRNA-transfection versus control transfections. α-Tubulin was used as loading control. ( e ) BrdU labelling indices were significantly decreased in Gabra2 siRNA-transfected pial ecs ( n =20, mean±s.d., * P <0.001, Student’s t -test). ( f ) sps explants showed chemoattraction (white arrows) to control siRNA-transfected pial ecs and this chemoattraction was reduced (yellow arrow) towards Gabra2 siRNA-transfected pial ecs. ( g , h ) Migration of control ( g ) and Gabra2 ( h ) siRNA-transfected pial ecs towards sps explant. Arrows show direction of migration. ( i ) Quantification of sps explant chemoattraction towards control and Gabra2 siRNA-transfected pial ecs ( n =25, mean±s.d., * P <0.0001, Student’s t -test). ( j ) Cell migration from sps explants was decreased when cultured on Gabra2 siRNA-transfected pial ecs. White arrows illustrate cell migration. ( k ) Quantification of migration assays of GE and sps explants on control and Gabra2 siRNA-transfected pial ecs ( n =20, mean±s.d., * P <0.0001, Student’s t -test, group ‘sps+control siRNA-transfected pial ecs’ compared with group ‘sps+ Gabra2 siRNA-transfected pial ecs’). ( l , m ) Co-labelled images of isolectin B4, GABA and DAPI labelling of control ( l ) and Gabra2 ( m ) siRNA-transfected pial ecs. ( n , o ) Individual isolectin B4, GABA and DAPI labelling of control ( n ) and Gabra2 ( o ) siRNA-transfected pial ecs ( × 60). ( p ) Gabra2 siRNA-transfected pial ecs failed to secrete GABA in contrast to control siRNA-transfected pial ecs ( n =6, mean±s.d., *** P <0.001, Student’s t -test). ( q – r ) Schema of GABA A receptors-GABA signaling in pv ecs (blue) and pial ecs (pink) that has consequences for deep (dark green) and superficial (light green) GABA neuron populations. GABA A receptors depicted as black ‘Y’ and GABA as yellow circles. ( a ) Scale bar, 40 μm; ( b ) scale bar, 13 μm; ( c ) scale bar, 28 μm; ( f ) scale bar, 100 μm (applies to g , h , j ); ( l ) scale bar, 50 μm (applies also to m ); and ( n ) scale bar, 15 μm (applies also to o ). Full size image The results of our studies are notable for several reasons. First, they reveal that preformed embryonic vascular networks are strategically positioned to fulfil the formidable task of providing support and guidance cues to GABA neurons on their lengthy tangential journey in the telencephalon. For the treatment of neurodegenerative diseases, a promising approach has been the transplantation of neuronal precursors into the adult brain. But, transplanted primary neuronal precursors have often been reported to remain at transplantation sites and are unable to migrate and integrate into regions that require new neurons [55] , [56] . This is usually explained by the absence of substrates to aid neuronal migration like radial-glial guides. The versatile pv ecs of the embryonic telencephalon may offer a solution for stalled neuronal precursors at transplantation sites. Second, they highlight the importance of endothelial cell diversity and function in the embryonic telencephalon and pave way to many important questions regarding specifically expressed genes in individual populations of endothelial cells based on their position in the CNS. Third, our results potentially implicate a new cell type-pv ecs as being contributory to a wide swath of neurological and psychiatric diseases. For example, the observation that many of the genes linked to schizophrenia are expressed in pv ecs will initiate future studies of this disease from a new perspective. In schizophrenia, multiple pathways in different cell types likely co-exist in patients synergistically inducing the highly complex form of this disease; and it is crucial to understand the autonomous program of these endothelial cells with respect to this disease. And finally, genes believed to independently regulate GABA neurogenesis and migration were expressed predominantly in pv ecs signifying that the periventricular angiogenesis gradient and GABA neuron developmental gradients are related to one another at mechanistic levels. The presence of GABA A receptors on periventricular and pial ecs and secretion of different levels of GABA by these populations of endothelial cells that has critical functions in attracting and promoting neuronal migration reveals a novel mechanism of GABA and its receptors’ signalling in the CNS ( Fig. 7q ). A role for GABA A receptor–GABA signalling in angiogenesis with consequences for GABA neuron migration opens new doors to pursue many questions in brain development and diseases that result from abnormal brain development like schizophrenia, epilepsy and autism. As we appreciate the new roles of periventricular angiogenesis, we begin also to encounter an important problem from another viewpoint. The problem is very significant indeed given that we have focused on neurological and psychiatric illnesses from a neuronal perspective extensively and it emphasizes the critical need to not underestimate the vasculature so intimately associated with neurons. The pioneering pv ecs of the telencephalon, that develop in advance of and free of neuronal development hold a valuable key for the establishment of the later forming neuronal networks and point to a novel paradigm of endothelial cell–neuron interactions in the embryonic forebrain. Animals Timed pregnant CD1 mice (E13) were purchased from Charles River laboratories, MA. Colonies of GAD65-GFP and Tie2-GFP mice were maintained in our institutional animal facility. The day of plug discovery was designated embryonic day 0 (E0). Animal experiments were in full compliance with the NIH Guide for Care and Use of Laboratory Animals and were approved by the McLean Institutional Animal Care Committee. Slice preparation and immunohistochemistry Brains from E13 GAD65-GFP embryos were collected and fixed in 4% paraformaldehyde at 4 °C. Vibratome slices (50 μm) were prepared and incubated in anti-biotinylated isolectin B4 (1:40, Sigma) with 1% TritonX-100 at 4 °C overnight. After six washes in PBS, slices were incubated with secondary antibody (Alexa 594 streptavidin conjugate) for 6 h at 4 °C. Flat mounted samples were analysed by a Zeiss LSM 5 Pascal laser confocal microscope. Images of the entire telencephalon were collected along the Z axis. The distance of GABA neurons to blood vessels was calculated from high-power Z-stack confocal images using ImageJ software. Embryonic brains from E13 CD1 mice were immersed in zinc fixative (BD Pharmingen) for 24 h and processed for paraffin histology. Double-labelling immunohistochemistry was performed on 20 μm thick paraffin-embedded sections with anti-biotinylated isolectin B4 (1:40, Sigma) and rabbit polyclonal anti-GAD65/GAD67 (Millipore, 1:400) antibodies. Secondary antibodies used were anti-rabbit Alexa fluor 488 conjugate and Streptavidin Alexa fluor 594 conjugate (Molecular Probes). Isolation and primary culture of endothelial cells E13 CD1 embryonic brains were dissected under a stereo-microscope and the telencephalon was removed. Pial membranes were peeled out and pooled (pial ecs). The remaining telencephalon without pial membranes was pooled as well (pv ecs). Mesencephalon and metencephalon were combined to prepare control endothelial cells. Purity of endothelial cell cultures was established with endothelial cell markers and determined to be a hundred per cent [5] . Isolation and culture of endothelial cells of the three sets were performed according to published methodology [5] . Chemoattraction and slice culture experiments In preparation for the chemoattraction assays, square culture inserts (ibidi Gmbh) were placed in the center of 35 mm collagen-coated culture dishes, to create a barrier (width - 0.9 cm). Cultures of periventricular and pial ecs were trypsinized and plated on either side of the barrier (experimental strategy outlined in text and Fig. 2b ). To prepare explants, GAD65-GFP+ve brains were cut at a thickness of 250 μm on a vibratome coronally. The GE region as well as subpial surface of ventral telencephalon (sps) were micro-dissected and further trimmed into blocks of equal size, respectively (All sps explant blocks were longer as they were isolated closely along the length of the subpial surface, whereas GE explant blocks were wider). Individual explants were plated in the barrier-free area of the plate with pial and pv ecs on either side. The co-culture was maintained for 24 h in FCS-DMEM (Invitrogen). At the end of the experiment, Tritc-conjugated isolectin B4 antibody (1:50, Sigma) was used to quickly label and visualize endothelial cells during subsequent imaging. The chemoattractive response of GFP+ve cells from the explant towards endothelial cells in each experiment were imaged and saved as JPEG files. In a parallel set of experiments, the same set of explants were plated on thin sheets of Geltrex basement membrane matrix (Invitrogen) that had been previously seeded with pial, periventricular or control endothelial cells. Following 12 h in vitro , the cultures were fixed in 4% paraformaldehyde and migration of GFP+ve cells were analysed. Images were taken and saved as TIFF files. The number and distance of migrating GFP+ve cells relative to the edge of the explant in all quadrants was calculated using ImageJ software and plotted. For disruption of pial and periventricular vascular networks, whole telencephalon explants prepared from E12 GAD65-GFP brains were transferred to polycarbonate membrane filters (8 μm pore size; Gibco-Life Technologies) in sterile six-well plates, incubated with Neurobasal medium (1 × , Gibco) and cultured for 36 h. For the bead experiments, heparin beads (Sigma) were washed thrice in PBS and soaked in angiogenesis inhibitor TNP-470 (Sigma, 10 μg) for 1–2 h at room temperature. Before implantation into the ventricular zone of the dorsal telencephalon, beads were washed in neurobasal medium. Control beads were treated identically with 0.1% BSA in PBS. To inhibit pial angiogenesis, 6-hydroxydopamine hydrochloride (6-OHDA, Sigma, 10 μg ml −1 ) was added to the culture medium. At the end of the experiment, explants were fixed in 4% paraformaldehyde, cryoprotected in sucrose gradient, embedded into frozen blocks and sectioned at 40 μm on a cryostat. Blood vessels were labelled with biotinylated isolectin B4 (1:40, Sigma) followed by secondary detection with Streptavidin Alexa fluor 594 conjugate. Dorsal telencephalon was imaged and images were saved as TIFF files. The density of GFP+ve cells in the selected areas was calculated from high magnification individual images using ImageJ software. Statistical significance of differences between groups in all sets of experiments was analysed by two-tailed Student’s t -test (Prism; GraphPad software). Fluorescence-activated cell sorting and RNA preparation Three sets of samples from E13 Tie2-GFP brains (in which endothelial cells express GFP specifically [5] ) are as follows: (1) Pial membranes from the telencephalon, (2) telencephalon without pia and (3) combined mesencephalon and metencephalon regions were individually minced into 1–2 mm fragments with a scalpel, rinsed in PBS and incubated at 37 ο C for 30 min in pre-warmed PBS with trypsin (0.25%), DNase I (1 mg ml −1 ) and EDTA (0.5 mM). Cells were dissociated, spun down, re-suspended in warm 10% FCS-DMEM and filtered through a sterile 100 μm nylon mesh. Cells were re-suspended in 1 ml RBC lysing buffer (Sigma), overlaid onto DMEM and centrifuged. Cells were washed with ice-cold FACS buffer (2% FCS and 0.1% NaN 3 in PBS) and incubated with Fcγ blocker (BD Biosciences, Pharmingen, 1 μg ml −1 ) for 30 min. Cells were washed in ice-cold FACS buffer and stained with anti-CD31 APC conjugated antibody (ebioscience) for 1 h. Cells were washed in ice-cold FACS buffer and GFP + /CD31 + endothelial cells were purified by fluorescence-activated cell sorting using a BD FACSAria-II flow cytometer (BD Biosciences, San Jose, CA). The gating parameters are slightly different because the experiments were performed at different days and the auto-fluorescence (background fluorescence) of the samples varied and the settings of the flow cytometer were different based on the background fluorescence. Thus, we gated in order to sort specifically GFP+ve population that were homogeneously expressing CD31 at a similar level. GFP fluorescence in purified endothelial cells was verified before RNA isolation. RNA was extracted from purified endothelial cells using the PicoPure RNA Isolation kit (Arcturus). RNA was shipped to Precision Biomarker Resources Inc, Evanston, IL where RNA quality was determined and microarray hybridization was performed. Gene expression profile analysis Affymetrix’s probe logarithmic intensity error (PLIER) signal of ‘15’ was used as the evidence of gene expression. The ratio of ‘periventricular’/‘pial’ ≥2.0 fold was arbitrarily considered as ‘periventricular’-favored gene activity and ‘pial’/‘periventricular’ ≥2.0 fold as ‘pial’-favored gene activity. The ratio of ‘periventricular’/‘control’ ≥2.0 fold was arbitrarily considered as ‘periventricular’-favored gene activity and ‘control’/‘periventricular’ ≥2.0 fold as ‘control’-favored gene activity. The lists of favored genes were subjected to a series of Enrichment GeneGo Ontology (Pathway Maps [57] , Biomarker-based Disease Category and Process Networks) as well as Go Processes and Go Molecular Functions analyses in MetaCore or literature survey for cell type-specific genes. The −log 10 ( P -value for significance) was used as enrichment score. ‘periventricular’ and ‘pial’ were analysed side by side and ‘periventricular’ and ‘control’ were analysed side by side for the sake of comparison unless indicated elsewhere. Real-time PCR RT was performed by using transcriptor first-strand cDNA synthesis kit (Roche Diagnostic). PCR reactions were run on an ABI Prism 7500 (Applied Biosystems) sequence detection system platform. Taqman primers with 6-carboxyfluorescein probe for Gabrb3 , Gabra1 , Cxcr4 , Cdk5r1 , Foxg1 and Sez6l2c were obtained from Applied Biosytems. The house keeping gene β2 microglobulin was used as a control. The relative gene expression among different samples and subsequent fold increase in periventricular versus pial ecs was determined according to published methodology [58] . Endothelial cell stainings and cell migration assays Periventricular and pial ecs were prepared from both CD1 and Tie2-GFP embryos. pv ecs were labelled with anti-GABRB3 (Sigma, 1:200) and pial ecs were labelled with anti-GABRA2 (Synaptic Systems, 1:400). Anti-biotinylated isolectin B4 (1:40, Sigma) was used for co-labelling and DAPI (Invitrogen) was used to label nuclei. Images were taken on an FSX100 microscope (Olympus). For siRNA transfections, pre-designed siRNA constructs for Gabrb3 , Gabra2 and a control non-targeting siRNA (Dharmacon) were used. Transfection of endothelial cells maintained at 80% confluency in six-well plates; cell harvest, lysis, blots and cell proliferation assays were performed according to published methodology [5] . Chemoattraction and migration assays were performed with transfected endothelial cells using similar methods described earlier. After 96 h of transfection, endothelial cells were processed for GABA immunohistochemistry (anti-GABA, Sigma, 1:400). Supernatants were also collected after 96 h of transfection and stored at −80 °C for ELISA. GABA concentrations were quantitatively determined by competitive ELISA according to manufacturers’ protocol (GABA Research ELISA kits, Labour Diagnostica Nord, Germany), and absorbance was measured using a multiplate microplate fluorescence reader (Molecular Devices, CA) at 450 nm. How to cite this article: Won, C. et al. Autonomous vascular networks synchronize GABA neuron migration in the embryonic forebrain. Nat. Commun. 4:2149 doi: 10.1038/ncomms3149 (2013).